Spin and orbital Ti magnetism at LaMnO3/SrTiO3interfaces In systems with strong electron-lattice coupling, such as manganites, orbital degeneracy is lifted, causing a null expectation value of the orbital magnetic moment. Magnetic structure is thus determined by spin–spin superexchange. In titanates, however, with much smaller Jahn–Teller distortions, orbital degeneracy might allow non-zero values of the orbital magnetic moment, and novel forms of ferromagnetic superexchange interaction unique to t 2g electron systems have been theoretically predicted, although their experimental observation has remained elusive. In this paper, we report a new kind of Ti 3+ ferromagnetism at LaMnO 3 /SrTiO 3 epitaxial interfaces. It results from charge transfer to the empty conduction band of the titanate and has spin and orbital contributions evidencing the role of orbital degeneracy. The possibility of tuning magnetic alignment (ferromagnetic or antiferromagnetic) of Ti and Mn moments by structural parameters is demonstrated. This result will provide important clues for understanding the effects of orbital degeneracy in superexchange coupling. The understanding and prediction of the collective responses exhibited by complex transition metal oxides is a major challenge of Condensed Matter sciences for the next decade [1] . Complexity in these materials results from a delicate interplay between lattice and spin-orbital-charge degrees of freedom [2] , [3] , [4] . In this framework and despite their common perovskite structures, titanates and manganites are electronically very different. In LaMnO 3 (LMO), with a d 4 electronic structure, the (spin up) t 2g band is fully occupied and there is a single electron in e g levels. The strong crystal field and electron–lattice Jahn Teller (JT) interactions lift orbital degeneracy, giving rise to an in-plane ordering of e g orbitals, which yields a ferromagnetic in-plane interaction, according to the Goodenough–Kanamori rules [5] , [6] . In titanates with a trivalent A site element, such as LaTiO 3 , Ti has a d 1 electronic configuration and thus there is a singly occupied t 2g band. The small crystal field splitting and the weak JT coupling (as compared with manganites with e g orbitals) result from the smaller overlap of t 2g orbitals (not directed along bond directions) with O π bonds. Owing to the nearly cubic environment of Ti ions, they exhibit a larger tendency to orbital degeneracy and may thus display orbital moments and low temperature ferromagnetism. However, there are important open questions such as the lack (or very small values) of the orbital moment [7] , [8] , [9] , [10] or the experimental absence of the ferromagnetism theoretically predicted for LaTiO 3 [11] , [12] . Modern thin-film growth techniques have succeeded in fabricating complex oxide heterostructures with atomically sharp interfaces, paving the way to interesting new phenomena. Electronic reconstruction [13] occurring at epitaxial interfaces [14] , [15] , [16] , [17] , [18] , [19] , [20] leads to the possibility of independently manipulating the essential quantities (electrostatic repulsion, hopping amplitude and doping), controlling electron correlations [1] , [2] and allowing the tailoring of their electronic response. This can be achieved in practice by manipulating the strained state [21] (permitting modification of orbital occupancy and ordering [2] ), or by controlling doping through suitable charge transfer processes resulting from differences in the electrochemical potential [22] . Moreover, the selection of materials with very different (or even antagonistic) ground states with controlled termination layers at the interfaces allows interactions to be tailored in a manner that may control competition and coupling of the order parameters [23] , [24] . Here we show that the combination of manganites and titanates in epitaxial heterostructures results in an exciting interfacial phenomenon. The titanate at the interface is doped as a result of a charge transfer process, and the Mn–O–Ti hybridized bonds offer a superexchange path for the magnetic coupling of Mn and Ti moments (see Fig. 1a ). The different orbital occupation of Mn depending on layer thickness ratio allows controlling the sign of this coupling (ferro- vs antiferromagnetic). 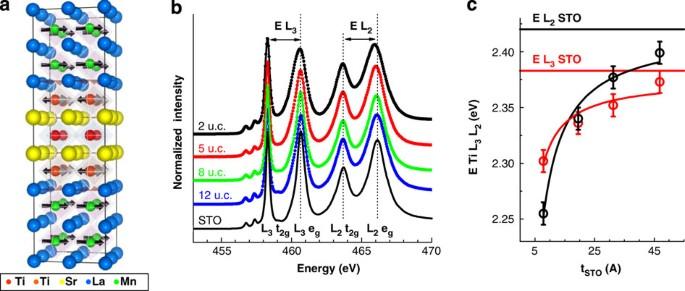Figure 1: X-ray isotropic absorption study of the titanate chemistry profile. (a) Schematic illustration of the LMO/STO heterostructures and a representative example of the magnetic structure arising at the interface. The colour code for the different ions is described at the bottom of the figure. Orange and red ions represent interfacial (electron doped) Ti and 'bulk' Ti4+ions, respectively. The black narrow arrows symbolize spin momentum, whereas the grey broad ones symbolize the orbital momentum. The oxygen of the ABO3perovskite structure has been removed for clarity. (b) Ti L2,3X-ray isotropic absorption spectra of (LMO 17/STO X) series of superlattices. The corresponding STO layer thickness can be consulted in the low-energy part of the figure. Line: STO substrate reference data. Data have been normalized to the height and position of the L3t2gpeak, and have been vertically shifted for clarity. (c) Energy difference between the egand t2gpeaks of the Ti L3(red open circles) and Ti L2(black open circles) absorption edges. The data have been plotted as a function of the STO layer thickness. The horizontal lines are the ΔEL3(red line) and ΔEL2(black line) experimental values of the STO substrate reference data. The curved lines are the experimental data fit result (see text). Error bars are the experimental energy resolution of ID08 (ESRF) beamline. Figure 1: X-ray isotropic absorption study of the titanate chemistry profile. ( a ) Schematic illustration of the LMO/STO heterostructures and a representative example of the magnetic structure arising at the interface. The colour code for the different ions is described at the bottom of the figure. Orange and red ions represent interfacial (electron doped) Ti and 'bulk' Ti 4+ ions, respectively. The black narrow arrows symbolize spin momentum, whereas the grey broad ones symbolize the orbital momentum. The oxygen of the ABO 3 perovskite structure has been removed for clarity. ( b ) Ti L 2,3 X-ray isotropic absorption spectra of (LMO 17/STO X) series of superlattices. The corresponding STO layer thickness can be consulted in the low-energy part of the figure. Line: STO substrate reference data. Data have been normalized to the height and position of the L 3 t 2g peak, and have been vertically shifted for clarity. ( c ) Energy difference between the e g and t 2g peaks of the Ti L 3 (red open circles) and Ti L 2 (black open circles) absorption edges. The data have been plotted as a function of the STO layer thickness. The horizontal lines are the Δ E L 3 (red line) and Δ E L 2 (black line) experimental values of the STO substrate reference data. The curved lines are the experimental data fit result (see text). Error bars are the experimental energy resolution of ID08 (ESRF) beamline. Full size image Materials growth and characterization We have grown LaMnO 3 /SrTiO 3 (LMO/STO) superlattices on (100) oriented STO single-crystalline substrates. In a previous paper [25] , we have shown that the interfaces are atomically sharp and free of defects, and thus we consider interdiffusion unlikely. Extended-emission-line spectrum, electron energy-loss spectroscopy (EELS) analysis with atomic resolution in an aberration-corrected scanning transmission electron microscopy has shown that the presence of an LaO plane at the interface with a donor character transfers electrons to the neighbouring TiO 2 planes. No evidence was found for further La inside the STO layer, which suggests that this LaO plane is not the result of an interdiffusion process. Multiple linear least-squares fits of the Ti absorption edge to reference spectra have shown a substantial amount of Ti 3+ at the interfacial TiO 2 plane, demonstrating that the interfacial plane functions as a La/Sr titanate chemically bonded to LMO. X-ray absorption spectroscopy In Figure 1b , the Ti L 2,3 isotropic X-ray absorption spectroscopy (XAS) measurements for the series of superlattices (LMO 17 unit cells (u.c. )/STO X u.c.) normalized to the L 3 t 2g edge jump and energy position are plotted. Compared with STO reference data (black line), all measurements display a similar sharp multiplet structure. It can be observed that the energy difference between the two main peaks of the L 3 and L 2 edges becomes smaller (as well as the width of the L 3 e g and L 2 e g peaks broadening) with the reduction of STO layer thickness. These results indicate the presence of Ti 3+ ions in the STO layers, and show that the concentration of Ti 3+ becomes higher as the STO layer thickness is reduced. As discussed in the next subsection, Ti 3+ atoms are located at the interface. To elucidate an approximate value for the average Ti oxidation state at the interface, we have fitted the energy difference between L 2 and L 3 peaks of Ti isotropic XA spectra to the equation where n T is the thickness of the STO layer (in unit cells, u.c. ), n 3+ is the number of Ti 3+ electron-doped unit cells and Δ E (L 2,3 ) STO and Δ E (L 2,3 ) LTO are the energy differences between e g and t 2g peaks of L 2 (Δ E (L 2 )) and L 3 (Δ E (L 3 )) spectral lines of bulk STO and LTO compounds, respectively (see Fig. 1b ). We deduce that only half a unit cell is electron doped; hence, the Ti oxidation state at the TiO 2 interface plane is approximately Ti 3.5+ . The fit (red and black curved lines in Fig. 1c ) makes use of the experimental values of Δ E (L 2,3 ) STO and the reported values of Δ E (L 2,3 ) LTO [26] . Previous scanning transmission electron microscopy–EELS measurements are also consistent with this result [25] . These electrons reside in the t 2g orbitals of a Ti band at the interfacial plane, which essentially functions as an 'artificially doped' interfacial titanate. The interfacial MnO 2 plane has an oxidation state close to 3+ (from EELS) with the 3 t 2g levels half-filled (because of Hund coupling) and one electron occupying the e g band. A substantial (5–10%) amount of holes in the manganite's conduction band, resulting either from interface charge transfer or from native stoichiometry defects, may be responsible for the robust ferromagnetism as revealed by magnetometry [25] . Interfacial strain has also been recently proposed to have an important role in producing ferromagnetism [27] . The electronic structure of the interface results from a combination of (doped) titanate and manganite, in which the presence of a Ti–O–Mn bond provides an exchange path between the 'magnetic' e g electrons of the manganite and nominally 'non-magnetic' t 2g electrons of the titanate, yielding an interesting magnetic response (see below). XMCD The electron-doped STO layers possess a magnetic moment, as clearly indicated by the presence of a strong XMCD signal. 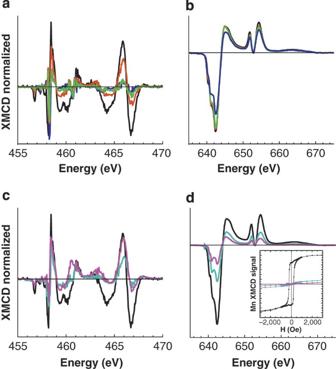Figure 2: Ti and Mn XMCD signals (6 K) for all samples. Ti (a)- and Mn (b)-normalized XMCD spectra of the series of superlattices with 17-u.c.constant LMO layer thickness and 2- (black), 5- (red), 8- (green) and 12 (blue)-u.c. STO layer thickness. Ti (c)- and Mn (d)-normalized XMCD spectra of the (LMO 3/STO 2) (magenta) and (LMO 7/STO 5) (cyan) superlattices compared with the (LMO 17/STO 2) (black) sample. The XMCD measurements are normalized to the L3t2g(Ti) and L3(Mn) edge-jump values. Inset: Mn hysteresis loops of the same samples obtained from Mn XMCD signal. In Figure 2 , the 6 K L 3 edge-jump-normalized XMCD signal for Ti and Mn of all superlattices can be observed. Two groups of samples have been examined in this study according to the LMO/STO thickness ratio. First, samples with constant LMO thickness (17 u.c.) changing the thickness of STO from 2 to 12 u.c. ( Fig. 2a and b ). These samples with thicker LMO than STO have a relaxed manganite and strained STO layers. In the second series ( Fig. 2c and d ), (LMO 7/STO 5) and (LMO 3/STO 2) samples have a thickness ratio corresponding to an optimally doped random alloy, but the reduced individual thickness of the layer results in an uniformly strained structure with the lattice parameters of the STO. The spectrum of the (LMO 17/STO 2) sample has also been included for comparison. The different strain patterns have been identified by X-ray diffraction experiments and can be found in the study by Garcia-Barriocanal et al . [25] Both sets of samples show the presence of Ti 3+ at the interface and XMCD spectra reveal a certain degree of Ti 3+ magnetism ( Fig. 2a and c ), aside from Mn magnetism ( Fig. 2b and d ). Note that for samples with constant LMO thickness ( Fig. 2a ), the Ti XMCD signal decreases by increasing the thickness of the top STO layer. This behaviour indicates that the Ti magnetism has an interfacial origin, as increase in STO layer thickness implies a reduction in the interfacial sensitivity. The Mn XMCD spectra series reveals a robust ferromagnetic moment of relaxed LMO layers ( Fig. 2b ) and a strong reduction of the ferromagnetic behaviour in samples with smaller LMO / STO thickness ratio with strained LMO layers ( Fig. 2d ). In fact, the Mn hysteresis loops obtained from XMCD measurements of strained LMO layers show very large saturation fields (essentially no saturation effects are observed up to 0.5 T) and do not show any coercive field, suggesting a possible (super)paramagnetic character (see inset of Fig. 2d ). Figure 2: Ti and Mn XMCD signals (6 K) for all samples. Ti ( a )- and Mn ( b )-normalized XMCD spectra of the series of superlattices with 17-u.c.constant LMO layer thickness and 2- (black), 5- (red), 8- (green) and 12 (blue)-u.c. STO layer thickness. Ti ( c )- and Mn ( d )-normalized XMCD spectra of the (LMO 3/STO 2) (magenta) and (LMO 7/STO 5) (cyan) superlattices compared with the (LMO 17/STO 2) (black) sample. The XMCD measurements are normalized to the L 3 t 2g (Ti) and L 3 (Mn) edge-jump values. Inset: Mn hysteresis loops of the same samples obtained from Mn XMCD signal. Full size image An important difference among the XMCD spectra of Figure 2c can be identified visually. It is clear that the magenta curve corresponding to the (LMO 3/STO 2) superlattice has a positive integral, whereas the black curve corresponding to the (LMO 17/STO 2) sample (with the same STO thickness) has a negative integral. This different XMCD shape reveals a different Ti?Mn interfacial magnetic coupling as discussed next. Although it is not possible to apply the sum rules to obtain a quantified value of the spin moments for the Mn and Ti ions, the XMCD integrals supply information about the relative size and orientation of both the observed spin and orbital moments of each cation. A detailed description of the application of the sum rules and the values of the orbital ( l Z ) and spin ( s Z ) moments from the integrals is described in the Methods section ( Fig. 4 ). Figure 4a and b display the integrated area under the XMCD spectra for Ti (a) and Mn (b) edges corresponding to two samples (LMO 17/STO 2 and LMO 3/STO 2) exhibiting the two extreme behaviours that are the subject of this study. 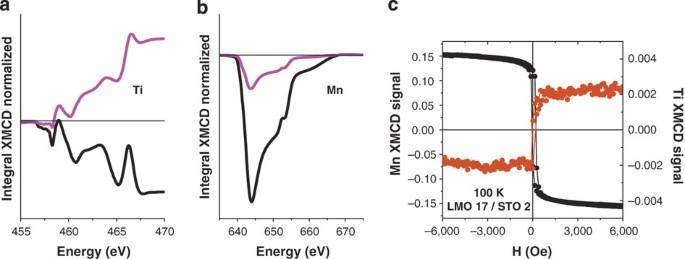Figure 4: Ferro- or antiferromagnetic coupling of Ti and Mn at the interfaces. Integrated values of the Ti (a)- and Mn (b)-normalized XMCD spectra of the (LMO 17/STO 2) (black) and (LMO 3/STO 2) (magenta) superlattices. The sample the magenta curve refers to has a relaxed STO layer and a strained LMO layer, the opposite is true for the black curve sample. (c) (LMO 17/STO 2) superlattice Ti (red) and Mn (black) hysteresis loops obtained from their XMCD signals at 100 K. Figure 4b shows a magnetic spin moment at the Mn edges in both samples, demonstrating that both samples are magnetic, as confirmed by magnetometry. Interestingly, although the integrals of the Mn XMCD spectra show that the orbital moment is essentially quenched as expected, there is a significant orbital component to the magnetic moment of the Ti (see Fig. 4a ). Note that the value of the Ti spin moment obtained from the application of the sum rules (0.2 μ B /Ti for (LMO 3/STO 2) and 0.15 μ B /Ti for (LMO 17/STO 2)) is to a great extent underestimated (see legends of the Fig. 4 ). Figure 4: Ferro- or antiferromagnetic coupling of Ti and Mn at the interfaces. Integrated values of the Ti ( a )- and Mn ( b )-normalized XMCD spectra of the (LMO 17/STO 2) (black) and (LMO 3/STO 2) (magenta) superlattices. The sample the magenta curve refers to has a relaxed STO layer and a strained LMO layer, the opposite is true for the black curve sample. ( c ) (LMO 17/STO 2) superlattice Ti (red) and Mn (black) hysteresis loops obtained from their XMCD signals at 100 K. Full size image The Ti spin moment estimated from the integrated XMCD spectra has a ferromagnetic character as illustrated by the Ti hysteresis loops displayed in Figure 4c . Note that the coercivity of the Ti loop is the same as that of the Mn. Furthermore, the temperature dependence of the Ti moment closely follows that of the Mn moment, and essentially vanishes at the Curie temperature of the manganite (see Supplementary Fig. S2 and Methods section), suggesting that the Mn–O–Ti superexchange is responsible for the Ti ferromagnetism in this sample. The shape of the XMCD signal of both Mn and Ti (see Fig. 4a and b ) depends strongly on the thickness ratio of the superlattices. Note that both samples display opposite signs of the integrated intensity under the Ti XMCD signal (see Fig. 4a ), clearly indicating a change in the coupling mechanism of the Ti and Mn spin moments at the interface. However, the size of the magnetic moment of the Ti does not scale with the Mn moment, which is reduced by more than a factor of 5 in the 3/2 sample as compared with the 17/2 (see Fig. 4b ). This suggests that, although magnetic alignment may be determined by superexchange, this mechanism alone does not explain the Ti spin magnetic moment. This is an important difference from the magnetism found at the Cu edge in cuprate/manganite interfaces, which has been shown to originate from spin canting of an otherwise AF spin structure of the cuprate at the interface, promoted by a ferromagnetic superexchange [23] . The plots of the integrals of the XMCD signals indicate that the orbital and spin moments of the Ti 3d electrons are in antiparallel alignment, evidencing the effect of spin orbit interaction. Spin-orbit coupling is a mechanism by which spins feel the distribution of the electronic density (orbits) and is described by a Hamiltonian of the form H SO = λ L·S. Spin-orbit coupling is different in e g and t 2g systems. For symmetry reasons, the matrix elements of the orbital momentum operator functioning on e g states are zero but are non-zero for t 2g states ( λ typically being 20 meV for titanates) [28] . Orbital magnetism is, on the other hand, expected in orbitally degenerate systems such as titanates. The unambiguous presence of an orbital moment antialigned to the spin constitutes direct evidence that the orbital degeneracy is not completely lifted (which would result in a complete quenching of the orbital moment). Antiparallel alignment of L and S moments is expected from Hund's third rule, assigning a positive value to the coupling constant λ and thus a minimum value of the J moment ( J = L – S ) to shells that, as is the case here, are less than half-filled. It is worthwhile recalling that experimental evidence in bulk LTO suggests that the orbital moment is almost completely quenched and no evidence of orbital magnetism has been found so far [10] , making our finding even more surprising and unexpected. X-ray linear dichroism Finally, we describe the relative alignment and possible magnetic coupling between Mn and Ti moments. In the (LMO 3/STO 2) superlattice (magenta line in the Fig. 4a ), the spin moments of interfacial Ti ions are ferromagnetically aligned with Mn spin moments. On the other hand, an antiferromagnetic alignment of the Ti and Mn spins moments is observed in samples with thicker LMO layers (LMO 17/STO 2) (black line in the Fig. 4a ). The different Ti–Mn interfacial magnetic couplings may be influenced by a different Mn e g orbital reconstruction promoted by the different strain or thickness patterns. Measurements of the XLD signal (see Fig. 5a ), and a further description in the Methods section and in Supplementary Fig. S3 , at room temperature evidence a change in the occupation of Mn orbitals at the interface. Manganese out-of-plane e g d(3z 2 -r 2 ) orbitals are occupied in (LMO 17/STO 2) samples with thick LMO layers (see Fig. 3b ), whereas the (LMO 3/STO 2) superlattices, with a much thinner manganite layer, promote a preferential in-plane e g d(x 2 –y 2 ) orbital occupation (see Fig. 5c ). This pattern of orbital occupation determined by epitaxial strain is in agreement with previous reports in ultrathin strained films [2] , [29] and modifies bonding in a way that may help to understand the sign of the superexchange interaction across the interface. Figure 5: Mn orbital occupation and magnetic interfacial couplings. 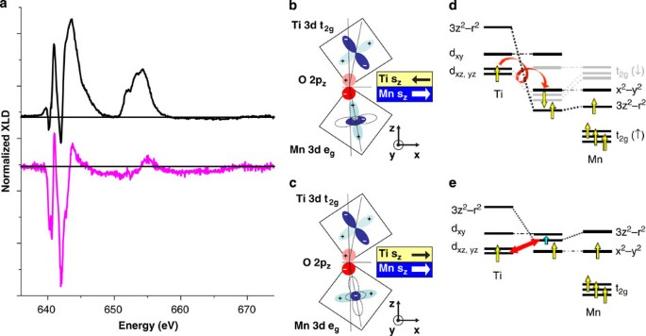Figure 5: Mn orbital occupation and magnetic interfacial couplings. (a) 300 K XLD of Mn normalized to the L3edge jump of the (LMO 17/STO 2) (black) and (LMO 3/STO 2) (magenta) superlattices. The sample the black curve refers to has a relaxed LMO layer, while the magenta curve refers to a sample with strained LMO layer. Sketches of the orbital occupation and magnetic couplings between Mn and Ti ions for the (LMO 17/STO 2) and (LMO 3/STO 2) superlattices are shown inFigure 5b and c,respectively. Note that in (b) the 3d(z2–r2) orbital is occupied, whereas in (c) the 3d(z2–r2) orbital is empty and the 3d(x2–y2) orbital is occupied instead. (d,e) Illustrate the possible schematic energy diagram arising at both interfaces. As a result of the different Mn orbital occupation, 4 (seed) and 3 (seee) bonding electrons participate in the hybridization process, giving rise to different Ti–Mn magnetic couplings. ( a ) 300 K XLD of Mn normalized to the L 3 edge jump of the (LMO 17/STO 2) (black) and (LMO 3/STO 2) (magenta) superlattices. The sample the black curve refers to has a relaxed LMO layer, while the magenta curve refers to a sample with strained LMO layer. Sketches of the orbital occupation and magnetic couplings between Mn and Ti ions for the (LMO 17/STO 2) and (LMO 3/STO 2) superlattices are shown in Figure 5b and c, respectively. Note that in ( b ) the 3d(z 2 –r 2 ) orbital is occupied, whereas in ( c ) the 3d(z 2 –r 2 ) orbital is empty and the 3d(x 2 –y 2 ) orbital is occupied instead. 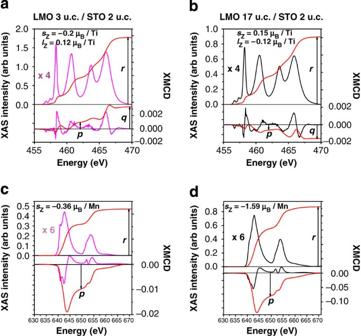( d , e ) Illustrate the possible schematic energy diagram arising at both interfaces. As a result of the different Mn orbital occupation, 4 (see d ) and 3 (see e ) bonding electrons participate in the hybridization process, giving rise to different Ti–Mn magnetic couplings. Figure 3: Sum rules forsZandlZ. Ti (a,b) and Mn (c,d) XAS and XMCD spectra of the samples (LMO3/STO 2) (magenta lines) and (LMO 17/STO 2) (black lines). The XA spectra have been corrected by the subtraction of a baseline that takes into account a linear increase of the background inside the L2,3edges, as well as the background out of the L2,3edge. The red lines are the integrated area of each signal. The orbital and spin moment of each cation can be consulted at the top of each figure. Arrows indicate the values ofp,qandr(see Methods). Full size image Figure 3: Sum rules for s Z and l Z . Ti ( a , b ) and Mn ( c , d ) XAS and XMCD spectra of the samples (LMO3/STO 2) (magenta lines) and (LMO 17/STO 2) (black lines). The XA spectra have been corrected by the subtraction of a baseline that takes into account a linear increase of the background inside the L 2,3 edges, as well as the background out of the L 2,3 edge. The red lines are the integrated area of each signal. The orbital and spin moment of each cation can be consulted at the top of each figure. Arrows indicate the values of p , q and r (see Methods). Full size image Semicovalent bonds at the interface result from the hybridization of d(3z 2 -r 2 ) and t 2g d(xz) and d(yz) active orbitals (both spin-up and spin-down). In the (LMO 17/STO 2) superlattice, there is strong hybridization between the preferentially occupied Mn d(3z 2 –r 2 ) band at the interface and the empty d(3z 2 –r 2 ) band of Ti. Hybridization of t 2g bands of Ti and Mn also occurs, although to a lesser degree because of the smaller overlap of t 2g orbitals. The occupation of the hybridized orbitals at the interface explains the AF alignment of the Ti moment with respect to the Mn moment [30] . Three of the electrons of the Mn occupy the spin-up d(3z 2 –r 2 ) and the active t 2g d(xz) and d(yz) hybrids, whereas the fourth occupies an inactive t 2g d(xy) orbital that does not participate in bonding. The Ti t 2g electron occupies the down-spin t 2g hybrid, and thus its alignment is antiferromagnetic (see Fig. 5d ). The dominant superexchange process occurs between the Ti t 2g electrons and the half-filled Mn t 2g bands and, according to Goodenough–Kanamori rules, is antiferromagnetic. In (LMO 3/STO 2) superlattices, the occupation of Mn d(x 2 −y 2 ) orbitals at the interface identified by X-ray linear dichroism (XLD) changes the hybridization pattern. The hybridization between the occupied Mn d(x 2 –y 2 ) and Ti orbitals across the interface is negligibly small. However, finite overlap between Ti t 2g and Mn d(3z 2 –r 2 ) orbitals may result from the GdFeO 3 -type distortion of the manganite observed in reciprocal space maps [25] . The sketches in Figure 5b and c indicate that, although the transfer integral between d(3z 2 –r 2 ) and t 2g active orbitals (d(xz) and d(yz)) is zero, a finite overlap results from the structural distortion. Ferromagnetic coupling in (LMO 3/STO 2) results from the superexchange interaction through the virtual excitation of electrons from Ti d(xz,yz) to Mn d(3z 2 –r 2 ). Alternatively, a charge transfer process suggested by the small values of the Mn magnetic moment obtained from XMCD and superconducting quantum interference device magnetometry and the larger ratio of Ti in a 4+ state obtained from EELS [24] and XAS may indicate a different scenario to explain the ferromagnetic coupling of the Ti moment. This charge transfer may result in partial occupancy of the d(3z 2 –r 2 ) bonding orbital as well, which provides a (ferromagnetic) Hund coupling to the Ti t 2g degenerate orbital, that is, the double-exchange interaction. The situation then is equivalent to having a fraction of spin-up electrons in t 2g antibonding orbitals resulting from the hybridization of Ti t 2g orbitals with the spin-up Mn t 2g band. We have shown that a simple molecular orbital picture, with mean-field-type treatment for the interaction, provides a simple explanation for the magnetic coupling of Ti and Mn moments at the interface. At this stage, we cannot make a definitive statement on the importance of corrections because of many-body effects or more complex spin-orbital superexchange processes not considered here. In summary, we have found evidence for Ti spin and orbital magnetism at the interface between an electron-doped titanate and a manganite. The orbital magnetic moment requires the presence of a small splitting between t 2g levels. This result constitutes a practical realization of orbital magnetism at an interfacial titanate layer that is not found in bulk titanates. Depending on the strain state of the superlattice, controlled by the manganite-to-titanate thickness ratio, the sign of the spin–spin coupling at the interface can be reversed, outlining the role of the orbital reconstruction at the interface in tailoring exchange interactions. This novel form of interface magnetism will provide important clues for understanding the effects of orbital degeneracy in superexchange coupling, and may have important practical implications in the operation of magnetic tunnel junctions in which spin polarization of the injected current may be influenced by the spin structure at the interface. Sample growth LMO/STO heterostructures were epitaxially grown on STO (001)-oriented substrates by means of a high-pressure pure oxygen (2.9 mbar) rf sputtering technique. Substrate temperature during growth was 810 °C. Superlattice samples consisted of eight repetitions of the bilayer (LMO X/STO Y), with X and Y in unit cells. Each sample started with an LMO layer grown on the STO substrate. Samples had good epitaxial properties, as confirmed by reciprocal space maps around in plane reflections. Details of the structural characterization of the samples can be found in study by Garcia-Barriocanal et al . [25] Magnetic circular dichroism XMCD X-ray absorption measurements with polarization dependence were determined at ID08 beamline of the European Synchrotron Radiation Facility and at the BL25SU beamline of SPring-8 at Japan, using a total electron yield detection method. Measurements were taken by tuning the X-ray beam at both the Mn and Ti L edges, with an incident beam angle of 70° with respect to the sample surface normal. Temperature was varied between 6 K and 300 K. The XMCD signal is the difference between absorption spectra obtained with plus and minus helicities of circular polarized light and supply elemental-specific information on magnetism. XMCD was recorded with an applied magnetic field of 1 T parallel to the X-ray beam direction (see Supplementary Fig. S1a ). Spin and orbital moments Spin and orbital moments can be obtained from XMCD spectra using sum rules [31] . However, it is well known that the 2p spin-orbit splitting of the light transition metal ions is not large enough to obtain accurate s z values from the sum rules. We have nevertheless used sum rules to determine a rough estimate of the order of magnitude and the relative orientation of the spin ( s Z ) and orbital ( l Z ) moments of Mn and Ti. The obtained s Z values are thus not accurate (in reality, they are usually underestimated). The l Z value, on the other hand, is obtained from the value of XMCD integral after the L 2,3 edge, and as this part of the spectrum is not affected by the small 2p spin-orbit splitting, the orbital moment as determined by sum rules is more accurate. Figure 3 displays the result of applying sum rules to Ti and Mn ions in samples (LMO 17/STO 2) and (LMO 3/STO 2). The s Z and l Z values obtained are also shown. Spin and orbital moments have been obtained from the following expressions: where n h is the number of holes in d shells (9 and 6 for Ti and Mn, respectively) and r is the integrated area of the isotropic XA spectra (we have considered that the isotropic XA spectra is the average of the spectra obtained with plus and minus helicities). q and p are the values of the integrated areas of the XMCD signal after the L 2,3 edge and between the L 3 L 2 edges, respectively (see Fig. 3 ). It is worth pointing out that Ti spin and orbital moments are antiparallely aligned, despite the same sign of p and q in the XMCD spectra. The antiparallel condition in XMCD measurements with the same sign of p and q is satisfied whenever the value of p is less than two-thirds of q . The following corrections have to be further taken into account to obtain the magnetic moments of Ti. As only Ti in a 3+ state contributes to the dichroic signal, whereas both Ti 3+ and Ti 4+ contribute to absorption, the ratio Ti 4+ /Ti 3+ has to be taken into account to correct for the active ions participating in the XMCD signal. A factor 6 has been used, as two STO unit cells contain three TiO 2 planes and only the half of the interfacial TiO 2 plane is electron doped, that is, only 50% of the interfacial Ti is in a 3+ state. The presence of interfacial Ti 3+ has been previously observed by atomic resolution EELS and later confirmed by the analysis of absorption spectra (see Results section). The second correction factor is the exponential attenuation of the XMCD signal. The magnetic interfacial Ti 3+ is buried below the surface of the STO top layer and its contribution to XMCD signal is thus attenuated by the inelastic scattering process that arises during the transport of the electron to the vacuum. A factor of 1.85 has been estimated considering the exponential decay of the Ti XMCD signal in the (LMO 17/STO X) series of samples, and assuming that the Ti magnetic moments are of the same magnitude in all of them. The temperature dependence of (3p–2q)- and q- normalized absolute values of both the Mn (red points) and Ti (black and green points) ions of (LMO 17/STO 2) superlattice obtained in a field-cooling (FC) 5T magnetic field is presented in Supplementary Figure S2 . The 1T FC superconducting quantum interference device measurement (black line) and XMCD data show a very similar trend. Mn and Ti spin and orbital moments display, within the experimental error, the same temperature dependence for the (LMO 17/STO 2) sample. The ferromagnetic alignment of the Ti spins seems to originate in an AF coupling to the ferromagnetic Mn spins at the interface. This idea is supported by the similar Ti and Mn coercitive fields exhibited by XMCD hysteresis loops obtained at Mn and Ti edges (see Fig. 4c ). Linear dichroism XLD XLD measurements were recorded at room temperature and were obtained from the difference of horizontal and vertical polarized light absorption spectra without applied magnetic field ( Supplementary Fig. S1b ). In these conditions, the XLD signal supplies a footprint of the orbital occupation of the different ionic species, free of the effect of magnetism, as the Curie temperature of all the samples of this study is always below room temperature [29] . XLD measures the excitation of core electrons to the unoccupied orbital. The linear dichroic signal results from the difference of the XAS spectra obtained with vertical linearly polarized light (VLP) and horizontal linearly polarized light (HLP) (see Supplementary Fig. S1 ). Note that, as the sample is mounted vertically, the convention to name VLP and HLP refers to in-plane (VLP) and out-of-plane (HLP). A preferential in-plane (VLP<HLP) or out-of-plane orbital occupation is deduced from the negative or positive (VLP>HLP) values of the XLD spectra (VLP–HLP), respectively. We have arrived at the conclusions sketched in Figure 5b and c of the paper as the Mn XLD spectra of the sample (LMO 17/STO 2) are positive (see Supplementary Fig. S3a ). This means that in-plane orbitals are less occupied and therefore the Mn e g electrons preferentially fill 3d(z 2 –r 2 ) orbitals. In contrast, in sample (LMO 3/STO 2), the XLD signal is negative, indicating a preferential occupation of the e g 3d(x 2 –y 2 ) orbitals, that is, there are more out-of-plane empty levels (see Supplementary Fig. S3b ). How to cite this article: Garcia-Barriocanal, J. et al . Spin and orbital Ti magnetism at LaMnO 3 /SrTiO 3 interfaces. Nat. Commun. 1:82 doi: 10.1038/ncomms1080 (2010).